The structural basis for selective binding of non-methylated CpG islands by the CFP1 CXXC domain CFP1 is a CXXC domain-containing protein and an essential component of the SETD1 histone H3K4 methyltransferase complex. CXXC domain proteins direct different chromatin-modifying activities to various chromatin regions. Here, we report crystal structures of the CFP1 CXXC domain in complex with six different CpG DNA sequences. The crescent-shaped CFP1 CXXC domain is wedged into the major groove of the CpG DNA, distorting the B-form DNA, and interacts extensively with the major groove of the DNA. The structures elucidate the molecular mechanism of the non-methylated CpG-binding specificity of the CFP1 CXXC domain. The CpG motif is confined by a tripeptide located in a rigid loop, which only allows the accommodation of the non-methylated CpG dinucleotide. Furthermore, we demonstrate that CFP1 has a preference for a guanosine nucleotide following the CpG motif. CpG islands contain a high density of CpG content and embrace the promoters of most genes in vertebrate genomes [1] . In the human genome, ∼ 70% of promoters have a high frequency of CpG dinucleotides. Generally, the CpG dinucleotides in the CpG islands of promoters are non-methylated, irrespective of transcription status of the associated genes, with some exceptions, such as those CpG islands associated with X chromosome and imprinted genes [2] . In spite of their conspicuous importance, the functional roles of the CpG islands in chromatin structure and transcription were unknown until recently. It has been shown that the CFP1 protein selectively binds non-methylated CpGs in vitro and in vivo [3] , consistent with previous studies, which showed that CFP1 binds non-methylated CpG motifs [4] , [5] . Furthermore, the non-methylated CpG islands (CGIs) coincide with sites of H3K4me3 in the mouse brain, and the H3K4me3 levels at CGIs were markedly reduced in CFP1-depleted cells [3] —this is not surprising considering the fact that CFP1 is a component of the histone H3K4 methyltransferase and binds the non-methylated CpG islands through its CXXC domain [3] , [6] , [7] , [8] . The study provided one of the first pieces of evidence that one major function of non-methylated CpG islands is to recruit chromatin-modifying complexes to modulate local chromatin structure through the CFP1- and CpG-island interactions. Blackledge et al . showed that CpG islands could directly recruit the H3K36-specific lysine demethylase enzyme KDM2A to create CpG island chromatin that is uniquely depleted of H3K36 methylation [9] . Similar to CFP1, KDM2A contains a CXXC domain that selectively recognizes non-methylated CpG motif and this binding is disrupted when the CpG sites are methylated [9] . The CXXC domain is found in a variety of chromatin-associated proteins and is characterized by two CGXCXXC repeats [10] . The CXXC domain contains eight conserved cysteine residues that bind two zinc ions and adopts an extended crescent-like structure [11] . In the human genome, there are over ten CXXC domain-containing proteins, and some of them have been shown to possess CpG-motif-binding ability in addition to CFP1 and KDM2A. For instance, the CXXC domain in mixed lineage leukemia (MLL) and its fusion proteins specifically recognizes non-methylated CpG DNA, and this interaction is essential for the recruitment of MLL to HoxA9 and leukemogenesis [11] , [12] , [13] , [14] , [15] , [16] , [17] . Methyl-CpG-binding domain (MBD) 1 contains three CXXC domains besides a MBD. The third CXXC domain in MBD1 binds specifically to non-methylated CpG, responsible for its methylation-independent localization [18] . Despite its important function, the molecular mechanism of the CXXC domain in selectively binding non-methylated CpG islands is unknown. Recently, a model for the CXXC domain of MLL and a CpG–DNA complex was proposed based on NMR spectroscopic data [13] , providing the first insight into how CXXC preferentially binds CpG DNA. Here we quantitatively compared the binding affinities of different CpG DNA with the CFP1 CXXC domain by isothermal titration calorimetry (ITC), and confirmed that CFP1 specifically binds to CpG DNA and prefers CpG DNA with a motif of CpGG. Furthermore, we determined a series of high-resolution crystal structures of the CFP1 CXXC domain in complex with CpG-containing DNA sequences. These structures elucidate the molecular mechanism of the non-methylated CpG-binding specificity by the CFP1 CXXC domain and why the CFP1 CXXC domain prefers a CpGG motif. CFP1 selectively binds CpG DNA with a preference for CpGG CFP1 is a component of the mammalian SETD1 complex and is essential for vertebrate development in different organisms [6] , [19] . Depletion of CFP1 gene causes a variety of developmental defects in zebra fish, murine and humans [8] , [19] , [20] . CFP1 has been shown to bind specifically to non-methylated CpG motifs through its CXXC domain and mutation of conserved residues in the CXXC domain caused loss of function [3] , [4] , [5] , [20] . By means of selected and amplified binding assay, it was found that the immediate flanking sequence around the CpG dinucleotide affects its binding with a preferred binding sequence of (A/C)CpG(A/C) [4] , [5] . To further characterize the binding selectivity of the CFP1 CXXC domain, we used electrophoretic mobility shift assay (EMSA) to analyse its DNA-binding ability. Our results show that all CpG-containing DNA oligonucleotides bind CFP1, and a DNA sequence with a GpC dinucleotide does not bind CFP1 ( Supplementary Fig. S1 ). Therefore, the CpG motif is essential for binding, consistent with previous reports [4] , [5] , [13] . In addition, to investigate how the flanking sequence surrounding the CpG dinucleotide affects CFP1 binding, we quantitatively measured the binding affinities of these CpG-containing DNAs by ITC assay. 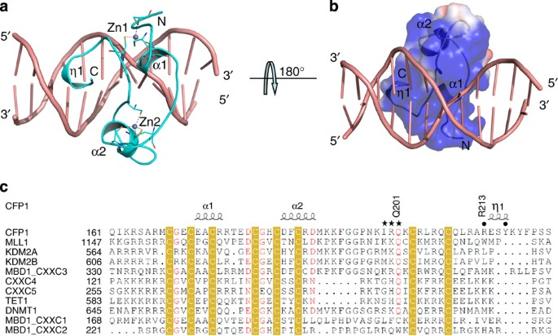Figure 1: Crystal structures of CFP1 in complex with a CpG DNA. (a) Cartoon representation of the crystal structure of human CFP1 CXXC domain in complex with a CpG DNA. The DNA and protein are coloured in salmon and cyan, respectively. (b) Electrostatic representation of the CFP1 CXXC domain in complex with a CpG DNA. The DNA is coloured in salmon. The secondary structure of the CFP1 CXXC domain is overlaid with the surface representation to assist in orientation. (c) Structure-based sequence alignment of CXXC domain of CXXC family members. The alignment was created with Espript (http://espript.ibcp.fr/ESPript/ESPript/). CFP1 (accession number: NP_055408): CFP1 CXXC domain; MLL1 (accession number: NP_005924): MLL1 CXXC domain; KDM2A (accession number: NP_036440): KDM2A CXXC domain; KDM2B (accession number: NP_115979): KDM2B CXXC domain; MBD1_CXXC3 (accession number: NP_056671): the third CXXC domain of MBD1; CXXC4 (accession number: NP_079488): CXXC4 CXXC domain; CXXC5 (accession number: NP_057547): CXXC5 CXXC domain; TET1 (accession number: NP_085128): TET1 CXXC domain; DNMT1 (accession number: NP_001370): DNMT1 CXXC domain; MBD1_CXXC1 (accession number: NP_056671): the first CXXC domain of MBD1; MBD1_CXXC2 (accession number: NP_056671): the second CXXC domain of MBD1. The eight conserved cysteines are coloured in yellow. Residues involved in recognition of CpG and the basepair following CpG are marked by stars and dots, respectively. Our binding data show that CFP1 has a modest preference for the CpGG trinucleotide-containing sequences ( Table 1 ). Table 1 Binding affinities of CFP1 to different CpG containing DNA sequences measured by ITC. 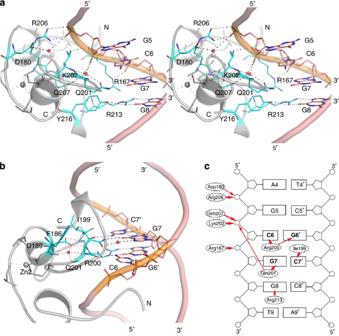Figure 2: Detailed interactions between the CFP1 CXXC domain and the GCGG double-stranded DNA (5′-GCCAGCGGTGGC-3′). (a) Stereo view of the interactions of the CFP1 CXXC domain with nucleotides outside the CpG motif. The DNA molecule and protein are coloured in salmon and grey cartoon representations, respectively. Residues or nucleotides involved in interactions are coloured in cyan sticks (CFP1) and salmon sticks (DNA). (b) CpG-specific interactions. The DNA molecule and CFP1 are coloured in salmon and grey cartoon representations, respectively. Residues or nucleotides involved in interactions are coloured in cyan sticks (CFP1) and salmon sticks (CpG). (c) Schematic representation of the CFP1 CXXC domain and the CpG–DNA complex. Hydrogen bonds, including those mediated by water, are marked by red arrows. Full size table CFP1 CXXC domain is wedged into the major groove of CpG DNA To better understand the molecular mechanism of selective binding of non-methylated CpG DNA by the CFP1 CXXC domain, we determined crystal structures of the CXXC domain of CFP1 (residues 161–222) in complex with six different CpG DNA sequences ( Table 2 ). Overall, these six complex structures are very similar. The CXXC domain of CFP1 consists of two alpha helices and one short 3 10 helix with two long loops linking them ( Fig. 1a–c ). Eight conserved cysteine residues bind two zinc ions to form two C4-type zinc fingers, with the first three cysteines and the last cysteine binding one zinc ion and the middle four cysteines binding the other zinc ion ( Fig. 1a,c ). The crescent-shaped CFP1 CXXC domain is wedged into the major groove of the CpG DNA and forms extensive interactions between the CXXC domain and DNA ( Fig. 1a,b ). The DNA-binding surface of CFP1 is predominantly positively charged, interacting with the negatively charged DNA ( Fig. 1b ). In addition to electrostatic interactions, a network of hydrogen bonds between the CXXC domain and DNA, including several water-mediated interactions, contribute to CFP1-DNA binding ( Fig. 2 ). Interestingly, only the middle four nucleotides including the CpG dinucleotide contribute to the CXXC binding. Table 2 Data collection and refinement statistics. Full size table Figure 1: Crystal structures of CFP1 in complex with a CpG DNA. ( a ) Cartoon representation of the crystal structure of human CFP1 CXXC domain in complex with a CpG DNA. The DNA and protein are coloured in salmon and cyan, respectively. ( b ) Electrostatic representation of the CFP1 CXXC domain in complex with a CpG DNA. The DNA is coloured in salmon. The secondary structure of the CFP1 CXXC domain is overlaid with the surface representation to assist in orientation. ( c ) Structure-based sequence alignment of CXXC domain of CXXC family members. The alignment was created with Espript ( http://espript.ibcp.fr/ESPript/ESPript/ ). CFP1 (accession number: NP_055408): CFP1 CXXC domain; MLL1 (accession number: NP_005924): MLL1 CXXC domain; KDM2A (accession number: NP_036440): KDM2A CXXC domain; KDM2B (accession number: NP_115979): KDM2B CXXC domain; MBD1_CXXC3 (accession number: NP_056671): the third CXXC domain of MBD1; CXXC4 (accession number: NP_079488): CXXC4 CXXC domain; CXXC5 (accession number: NP_057547): CXXC5 CXXC domain; TET1 (accession number: NP_085128): TET1 CXXC domain; DNMT1 (accession number: NP_001370): DNMT1 CXXC domain; MBD1_CXXC1 (accession number: NP_056671): the first CXXC domain of MBD1; MBD1_CXXC2 (accession number: NP_056671): the second CXXC domain of MBD1. The eight conserved cysteines are coloured in yellow. Residues involved in recognition of CpG and the basepair following CpG are marked by stars and dots, respectively. Full size image Figure 2: Detailed interactions between the CFP1 CXXC domain and the GCGG double-stranded DNA (5′-GCCAG CG GTGGC-3′). ( a ) Stereo view of the interactions of the CFP1 CXXC domain with nucleotides outside the CpG motif. The DNA molecule and protein are coloured in salmon and grey cartoon representations, respectively. Residues or nucleotides involved in interactions are coloured in cyan sticks (CFP1) and salmon sticks (DNA). ( b ) CpG-specific interactions. The DNA molecule and CFP1 are coloured in salmon and grey cartoon representations, respectively. Residues or nucleotides involved in interactions are coloured in cyan sticks (CFP1) and salmon sticks (CpG). ( c ) Schematic representation of the CFP1 CXXC domain and the CpG–DNA complex. Hydrogen bonds, including those mediated by water, are marked by red arrows. Full size image The overall structure of the CFP1 CXXC domain resembles the recently reported structure of the MLL CXXC domain [13] ( Fig. 3a,b ). The major differences between these two CXXC domain structures are at the amino (N)- and carboxy (C)-termini ( Fig. 3c ). Both N- and C-termini of the CXXC domain extend into a minor groove of the CpG DNA in the MLL–DNA complex structure [13] ( Fig. 3a ). In contrast, the C-terminus of the CFP1 CXXC domain forms a short 3 10 helix and interacts only with the major groove of DNA ( Figs 1a and 3b ). The first α-helix (α1) of the CFP1 CXXC domain hangs over the DNA backbone with the preceding loop extending into the minor groove but not making direct contact with DNA ( Figs 1a and 3b ). Hence, the CFP1 CXXC–DNA contacts are all with the major groove of the DNA, consistent with the DNA perturbation analysis of the MLL CXXC domain [11] . On the other hand, when we superimposed the CXXC domains of CFP1 and MLL together, we found that there is a significant shift between the DNA helices in these two CXXC–DNA complex structures ( Fig. 3c ). The NMR MLL CXXC–DNA complex structure used a canonical B-form DNA for modelling the complex structure [13] . However, on the basis of our crystal complex structures, we found that the major groove of the CpG DNA is distorted and 2.0 Å wider than that of a canonical B-form DNA, because of the insertion of the CFP1 CXXC domain ( Fig. 3d ). We also compared the two DNAs with the CFP1 and MLL complexes and found that the former has a 3.4 Å wider major groove than the latter ( Supplementary Fig. S2 ). During the revision of this manuscript, the crystal structure of DNMT1–DNA complex was reported [21] . In this structure, the CXXC domain is also inserted into the major groove of the CpG DNA and causes the major groove widening ( Supplementary Fig. S3 ). 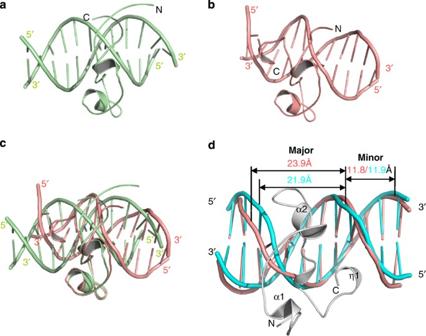Figure 3: Comparison of CFP1–CpG complex (CCGG1) with MLL1–CpG complex (PDB id: 2KKF). (a) Overall structure of MLL1-CpG DNA shown in green cartoon representation. (b) Overall structure of CFP1-CpG DNA shown in salmon cartoon representation. (c) Superposition of the CFP1 CXXC domain (salmon) and the MLL1 CXXC domain (green) of the MLL–DNA and CFP1–DNA complexes. (d) Superimposition of the CpG DNA from the CFP1–DNA complex (salmon) and the standard 12-mer B-form DNA (cyan; PDB id: 1HQ7). The protein is shown in grey cartoon representation. The widths of major grooves and minor grooves of both DNAs are marked in red (CFP1 DNA) and cyan (B-DNA), respectively. Figure 3: Comparison of CFP1–CpG complex (CCGG1) with MLL1–CpG complex (PDB id: 2KKF). ( a ) Overall structure of MLL1-CpG DNA shown in green cartoon representation. ( b ) Overall structure of CFP1-CpG DNA shown in salmon cartoon representation. ( c ) Superposition of the CFP1 CXXC domain (salmon) and the MLL1 CXXC domain (green) of the MLL–DNA and CFP1–DNA complexes. ( d ) Superimposition of the CpG DNA from the CFP1–DNA complex (salmon) and the standard 12-mer B-form DNA (cyan; PDB id: 1HQ7). The protein is shown in grey cartoon representation. The widths of major grooves and minor grooves of both DNAs are marked in red (CFP1 DNA) and cyan (B-DNA), respectively. Full size image In addition, it was reported that the N-terminus of the MLL CXXC domain is involved in DNA binding and enhances binding [13] . However, we noticed that the N-terminus (residues 1,147–1,151) of the MLL CXXC domain is not well converged in the 20 NMR models of the MLL CXXC–DNA complex. The Arg1150 is shown to contact the DNA backbone in some conformations, but points to the solvent in other conformations. This kind of divergence among different conformations also exists in other N-terminal residues, such as Arg1151 and Ser1152. Therefore, the N-terminus of the MLL CXXC domain is very flexible and does not form stable interactions with the CpG DNA. Similarly, in our complex structure, the corresponding N-terminus does not contact DNA directly, although it hangs over a minor groove of the CpG DNA. To explore whether the fragment N-terminal to the CFP CXXC domain is involved in DNA binding, we made a longer CFP1 construct (residues 152–222) and tested whether the extended CFP1 CXXC domain would bind DNA more tightly. Our results indicate that the longer construct only binds CpG DNA with a slightly greater affinity than the shorter construct ( Table 3 ), indicating that the extended N-terminal fragment of the CFP1 CXXC domain may not contribute significantly to the DNA binding. Table 3 Binding affinities of the CpG DNA (CCGG1: 5′-GCCAC CG GTGGC-3′) to different CFP1 mutants and the first CXXC domain of MBD1. Full size table Structural basis of CpG-specific recognition by CFP1 CXXC domain has been shown to specifically recognize non-methylated CpG motif by selected and amplified binding, EMSA and quantitative ITC assays [4] , [5] , [11] , [13] . Our high-resolution complex structures of the CFP1 CXXC domain and DNA provide the molecular basis for understanding this specificity. The CpG motifs from the DNA duplex are selectively recognized by the CFP1 CXXC domain through six base-specific hydrogen bonds ( Fig. 2b ). The two guanosines G6′ and G7 each form two hydrogen bonds with the side chain of R200 (G6′) and the side chain of Q201 and a conserved water molecule (G7), respectively. The two cytosines C7′ and C6 each form a hydrogen bond with the backbone carbonyl oxygen of I199 and R200 through their N4-amine groups, respectively ( Fig. 2b ), which is consistent with the recently published NMR complex structure of MLL CXXC domain with DNA [13] . Substituting either cytosine for adenosine or guanosine will disrupt the hydrogen bond, whereas replacing cytosine for thymidine or methylating the C5 atom of cytosine will cause a steric clash with the protein backbone. Hence, the CpG is tightly bound by the I199–R200–Q201 tripeptide. Most importantly, the IRQ tripeptide is located in a very rigid loop linking the second α2 helix and the C-terminal 3 10 helix. The IRQ tripeptide is packed against the α2 helix and forms two hydrogen bonds with D189 and one hydrogen bond with F186 through a conserved water molecule. Both D189 and F186 are located on the α2 helix. The IRQ loop and the α2 helix are also held together by the second Zn ion. Therefore, this CpG recognition loop is tightly fastened in the CXXC domain and is unable to undergo conformational changes to accommodate methylated CpG or other sequences. Interestingly, Q201 is highly conserved in the CXXC domains ( Fig. 1c ), and its importance is confirmed by mutagenesis binding measurement. Mutating Q201 to alanine abolishes binding ( Table 3 ). In addition, on the basis of sequence alignment, we found that the corresponding residue to Q201 in the first CXXC domain of MBD1 is a cysteine. Consistently, the first CXXC domain of MBD1 lacks CpG DNA-binding ability ( Table 3 ). The non-methylated CpG-binding mode adopted by CXXC domain is markedly different from that adopted by the MBD domain or SRA domain, which preferentially bind fully methylated or hemi-methylated CpG DNA, respectively [22] , [23] , [24] , [25] ( Supplementary Fig. S4 ). The MBD domain in methyl CpG binding protein 2 (MECP2) recognizes the hydration of the major groove of fully methylated CpG [22] ( Supplementary Fig. S4a ), whereas the SRA domain in UHRF1 (Ubiquitin-like, containing PHD and RING finger domains 1) accommodates base-flipped 5-methylcytosine in a binding pocket with planar stacking, hydrogen bond and van der Waals interactions [23] , [24] , [25] ( Supplementary Fig. S4b ). Preferential binding of CFP1 CXXC domain to the CpGG motif From the comparison of these six CFP1–DNA complex structures, we could also gain insight into why the CFP1 CXXC domain prefers a guanosine nucleotide following the CpG dinucleotide. Among these six complex structures, the major structural difference lies on how R213 interacts with the base of the nucleotide following the CpG dinucleotide. In the complex structures of CFP1 with the CpGG DNA, G8 base forms two hydrogen bonds with R213 ( Figs 2a and 4a ). However, in the complex structure of CFP1 with the CpGT DNA, the hydrophobic C5 methyl group (C5M) of the thymidine T8 pushes away the positively charged R213 side chain and disrupts the hydrogen bonds ( Fig. 4a ). Similarly, in the case of the CFP1–CpGA DNA complex, the NH2 group at the N6 position of adenosine A8 also pushes away the side chain of Arg213 ( Fig. 4b ). We could not get crystals of the CFP1–CpGC complex, maybe because of the low binding affinity between CFP1 and the CpGC DNA ( Table 1 ). Nevertheless, we built a model for the CFP1–CpGC complex ( Fig. 4c ), which shows that the NH2 group at the N4 position of C8 would also push Arg213 away, analogous to the CpGT case. In all these three cases, R213 side chain reorients and is brought close to the side chain of R167, which is not energetically favourable because of the electrostatic repulsion. This observation is consistent with our binding results, that is, when the guanosine in the CpGG motif is replaced by T, A or C, the binding affinity of DNA to the CFP1 CXXC domain is reduced by 4–8-folds ( Table 1 ). Furthermore, mutating R213 to alanine also diminished the binding of CFP1 to the CpG DNA significantly (>60-fold; Table 3 ), which indicates that the non-CpG-specific interaction also has an important role in the formation of the complex. The binding affinity of another CFP1 mutant, Y216A, is reduced by more than fourfolds ( Table 3 ). In our complex structure of the CFP1 and CpGG, Y216 is hydrogen bonded to the side chain of R213 to stabilize R213 and facilitate the recognition of G8 by R213 ( Figs 2a and 4a ). In all non-CpGG complexes, the hydrogen bond between Y216 and R213 is disrupted ( Fig. 4 ). 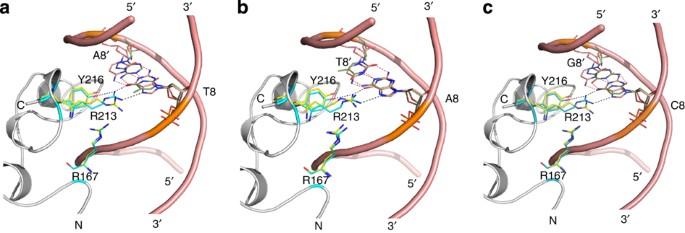Figure 4: CFP1 preferentially binds CpGG trinucleotide. (a) Superposition of CpGT with CpGG complexes. (b) Superposition of CpGA with CpGG complexes. (c) Superposition of CpGC with CpGG complexes. The DNA molecule and protein are coloured in salmon and grey cartoon representations, respectively. The DNA basepairs following the CpG dinucelotide are coloured in salmon (CpGG) and green sticks (the other three), respectively. R167 and R213 and Y216 are coloured in cyan (CpGG) and yellow (the other three) sticks, respectively. Figure 4: CFP1 preferentially binds CpGG trinucleotide. ( a ) Superposition of CpGT with CpGG complexes. ( b ) Superposition of CpGA with CpGG complexes. ( c ) Superposition of CpGC with CpGG complexes. The DNA molecule and protein are coloured in salmon and grey cartoon representations, respectively. The DNA basepairs following the CpG dinucelotide are coloured in salmon (CpGG) and green sticks (the other three), respectively. R167 and R213 and Y216 are coloured in cyan (CpGG) and yellow (the other three) sticks, respectively. Full size image Although the nucleotide preceding the CpG dinucleotide also interacts with the CFP1 CXXC domain, the nucleotide substitution at this position does not affect binding ( Table 1 ). From the complex structures, we can see that the nucleotide contacts CFP1 mainly through the backbone ( Fig. 2c ). In this study, we utilized X-ray crystallography and quantitative ITC-binding assay to systematically study the binding selectivity of the CFP1 CXXC domain. Our binding results show that the CFP1 CXXC domain binds any CpG-containing DNA with a preference for the CpGG motif. Our high-resolution complex structures demonstrate that CFP1 uses a rigid IRQ tripeptide to selectively bind the CpG dinucleotide, and uses the R213 and to a lesser extent Y216 residues to discriminate the CpGG motif over CpGT, CpGA and CpGC motifs. Recently, an NMR model of the MLL CXXC domain with a CpG DNA was proposed [13] , assuming that the DNA adopts a canonical B-form conformation. Our structures show that the DNA is distorted because of the insertion of the CFP1 CXXC domain into the major groove of the CpG DNA. When we superimposed these two CXXC domain complex structures based on the CXXC domain, we found that there exists a three-base shift at one end of the two DNAs ( Fig. 3c ). When we compared the DNA in the CFP1 complex with a canonical DNA or the DNA from the MLL complex, we observed a 2.0 and 3.4 Å widening in the major groove of the CFP1 DNA ( Fig. 3d and Supplementary Fig. S2 ). Thus, it is possible that the CpG DNA in the MLL CXXC–DNA complex is also distorted upon binding to the MLL CXXC domain, although we could not exclude the possibility that different CXXC domain display different binding modes, which needs to be further investigated in the future. Another major discrepancy between the CFP1 and MLL CXXC domains is that a short 3 10 helix (η1) is formed in the C-terminus of the CFP1 CXXC domain ( Fig. 1a ). We have identified that R213 and Y216 are two important residues in determining the binding preference of CFP1 for the CpGG motif. Interestingly, Y216 is located in that 3 10 helix and R213 is just preceding the C-terminal 3 10 helix ( Fig. 1c ). On the basis of the structure-based sequence alignment ( Fig. 1c ), we found that the 3 10 helix sequence is not conserved in other CXXC family members, therefore, the CpGG sequence preference may not hold for other members of the CXXC family, which may have different binding preferences. CFP1 is a component of the H3K4 methyltransferase SETD1 [6] . Another H3K4 methyltransferase MLL contains a CpG-binding CXXC domain, which is essential for the recruitment of MLL to HoxA9 and leukemogenesis [11] , [12] , [13] , [14] , [15] , [16] , [17] . The CXXC domain in the histone H3K36 demethylase KDM2A is proved to bind CpG DNA and recruit its histone demethylation activity to its target genes [9] . Thus, the CXXC domain could function as a recruiting element directing different chromatin-modifying activities to various chromatin domains to regulate local chromatin structure and gene expression, in addition to providing a possible mechanism to keep these CpG islands methylation-free and antagonize abnormal gene silencing and disease [3] , [9] . Our observation that CFP1 preferentially binds a CpGG motif might implicate that the CXXC domain would have an important role in targeting its associated activities to specific target genes by selectively binding different CpG islands located in the promoters of these target genes through the diverse CXXC domains. Protein expression and purification The human CFP1 CXXC domain (residues 161–222) was subcloned into pET28a-MHL vector. The recombinant protein was over-expressed at 18 °C as an N-terminal His6-tagged protein in E. coli BL21 (DE3) Codon plus RIL (Stratagene) and was purified by HiTrap Ni column and Superdex 75 gel-filtration column. The protein was concentrated to 10 mg ml −1 in a buffer containing 20-mM Tris, pH 7.5, 0.15-M NaCl, 1-mM DTT and 50-μM ZnCl 2 . Isothermal titration calorimetry Isothermal titration calorimetry measurements were recorded at 25 °C using a VP-ITC microcalorimeter (MicroCal Inc.). Experiments were performed by injecting 10 μl of DNA solution (0.5–1 mM) into a sample cell containing 15–100 μM of CFP1 CXXC domain protein (wild type or its mutants) in 20-mM Tris-HCl, pH 7.5, 150-mM NaCl, 1-mM DTT and 50-μM ZnCl 2 . Different DNA oligos were dissolved and dialysed into the same buffer as that of the CPF1 CXXC domain protein. The concentrations of proteins and DNAs are estimated with absorbance spectroscopy using the extinction coefficient, OD 280 and OD 260 , respectively. A total of 27 injections were performed with a spacing of 180 s and a reference power of 13 μcal s −1 . Binding isotherms were plotted and analysed using Origin Software (MicroCal Inc.). The ITC measurements were fit to a one-site binding model. EMSA Ready gels are purchased from Bio-Rad Laboratories, Inc. The running buffer is 0.5× TBE (Tris/Borate/EDTA) made from 10× TBE stock. The concentration of each double-stranded DNA is 50 μM and is mixed with protein in a 1:5 molar ratio. The gel is stained by ethidium bromide staining. Protein crystallization All DNAs are purchased from Integrated DNA Technologies, Inc. Before using for crystallization, each pair of single-strand DNAs is mixed in a 1:1 molar ratio, and then heated and annealed to form double-stranded DNA. For cocrystallization, purified CFP1 CXXC protein was mixed with different CpG DNAs at a molar ratio of 1:1.2 and then crystallized using the hanging drop vapour diffusion method at 18 °C. CFP1 and CpG DNA was crystallized in a buffer containing 0.1-M Hepes sodium, pH 7.5, 0.2-M CaCl 2 , 28% PEG 400 (GCGG, CCGG1 and ACGG DNAs) or 0.1-M Hepes sodium, pH 7.5, 0.1-M MgCl 2 , 30% 550 MME (TCGT, ACGT and TCGA DNAs). Before flash-freezing crystals in liquid nitrogen, crystals were soaked in a cryoprotectant consisting of 100% reservoir solution and 12% glycerol. Structure determination The structure of human CXXC1-CCGG1 DNA was solved using the single-wavelength anomalous dispersion method [26] , [27] utilizing the anomalous signal from Zn ions present in the crystals. To maximize the anomalous signal, diffraction data were collected at 100 °K on beamline 19-ID (Structural Biology Centre, Advanced Photon Source, Argonne National Laboratory) at the peak wavelength of the Zn–K absorption edge (1.2832 Å), and data were integrated and scaled using the HKL2000 software package [28] . The positions of two Zn anomalous scatterers were determined using SHELXD [29] , followed by heavy-atom refinement and maximum likelihood-based phasing as implemented in the autoSHARP program suite [30] . Phase improvement by density modification generated an interpretable experimental electron density map, which allowed an initial model of the polypeptide chain to be traced using ARP/warp [31] . Following several alternate cycles of restrained refinement against a maximum likelihood target and manual rebuilding using COOT [32] , the improved model revealed clear electron densities allowing placement of the bound double-stranded CpG oligonucleotide (CCGG1). All refinement steps were performed using REFMAC [33] . The final model was refined against a high-energy remote data set collected at higher resolution with a second crystal on beamline 19-ID. The remaining DNA-bound CXXC1 structures (GCGG, TCGT, ACGT, TCGA and ACGG complexes) were subsequently solved by molecular replacement method as implemented by MOLREP in the CCP4 program suite [34] using the CXXC1/CCGG1 structure as a search model. Model improvement was achieved through several alternate cycles of restrained refinement and manual rebuilding. During the final cycles of model building, translation-libration-screw (TLS) parameterization [35] was included in the refinement of all models, which comprised of protein, DNA and solvent molecules. Data collection and refinement statistics are summarized in Table 2 . Accession codes: Atomic coordinates and structure factors for the CFP1 CXXC domain in complex with the six CpG DNAs have been deposited in the Protein Data Bank under the accession codes 3QMB , 3QMC , 3QMD , 3QMG , 3QMH , 3QMI . How to cite this article: Xu, C. et al . The structural basis for selective binding of non-methylated CpG islands by the CFP1 CXXC domain. Nat. Commun. 2:227 doi: 10.1038/ncomms1237 (2011).